Construction of C-B axial chirality via dynamic kinetic asymmetric cross-coupling mediated by tetracoordinate boron 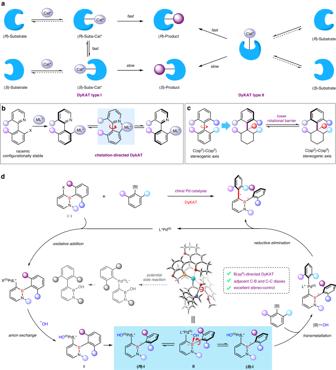Fig. 1: Previous transition-metal-catalyzed atroposelective cross-coupling reactions and our reaction design. aDynamic kinetic asymmetric transformation (DyKAT).bChelation-directed DyKAT of racemic heterobiaryls.cC(sp2)−C(sp3) axial chirality.dA tetracoordinate boron-directed DyKAT to access the challenging atropisomers bearing C-B stereogenic axis, or adjacent C-B and C-C diaxes (this work). Catalytic dynamic kinetic asymmetric transformation (DyKAT) provides a powerful tool to access chiral stereoisomers from racemic substrates. Such transformation has been widely employed on the construction of central chirality, however, the application in axial chirality remains underexplored because its equilibrium of substrate enantiomers is limited to five-membered metalacyclic intermediate. Here we report a tetracoordinate boron-directed dynamic kinetic asymmetric cross-coupling of racemic, configurationally stable 3-bromo-2,1-azaborines with boronic acid derivatives. A series of challenging C-B axially chiral compounds were prepared with generally good to excellent enantioselectivities. Moreover, this transformation can also be extended to prepare atropisomers bearing adjacent C-B and C-C diaxes with excellent diastereo- and enantio-control. The key to the success relies on the rational design of a reversible tetracoordinate boron intermediate, which is supported by theoretical calculations that dramatically reduces the rotational barrier of the original C-B axis and achieves the goal of DyKAT. Catalytic dynamic kinetic asymmetric transformation (DyKAT) has emerged as a powerful platform for 100% theoretical conversion of racemic, configurationally stable substrates into high-value optically pure compounds [1] , [2] like numerous pharmaceuticals and natural products [3] , [4] , [5] , [6] . Mechanistically, these reactions normally entail a chiral catalyst-mediated equilibration of substrate enantiomers, involving formation of diastereomeric substrate−catalyst intermediates with unstable configuration (DyKAT type I, Fig. 1a ) or a common chiral intermediate that has lost the substrate’s chiral center (DyKAT type II, Fig. 1a ). DyKAT strategy has been widely employed on central chirality [2] , in recent years, it has also demonstrated important applications on the construction of heterobiaryl atropisomers [7] , which are prevalent in natural products, medicines, ligands, catalysts and materials [8] , [9] , [10] , [11] , [12] , [13] , [14] , [15] , [16] , [17] . The transition-metal-catalyzed DyKAT of racemic, configurationally stable heterobiaryl substrates have been applied in the synthesis of axially chiral heterobiaryl compounds [18] , [19] , [20] , [21] , [22] , [23] , [24] , [25] since the pioneering works by Lassaletta & Fernandez [18] and Virgil & Stoltz [19] . The key of these elegant works all depends on the fast interconversion of diastereomeric substrate−catalyst intermediates promoted by five-membered metalacyclic intermediates [18] , [19] , [20] , [21] , [22] , [23] , [24] , [25] (Fig. 1b ). However, the monotonous reaction mode significantly restricts the wide application of DyKAT on axial chirality, and the challenge is to explore and find more modes to promote equilibrium of substrate enantiomers. Fig. 1: Previous transition-metal-catalyzed atroposelective cross-coupling reactions and our reaction design. a Dynamic kinetic asymmetric transformation (DyKAT). b Chelation-directed DyKAT of racemic heterobiaryls. c C( sp 2 )−C( sp 3 ) axial chirality. d A tetracoordinate boron-directed DyKAT to access the challenging atropisomers bearing C-B stereogenic axis, or adjacent C-B and C-C diaxes (this work). Full size image Compared with the common C( sp 2 )−C( sp 2 ) atropisomers, the C( sp 2 )−C( sp 3 ) atropisomers have a lower rotational barrier because the conical space of sp 3 carbon is more conducive to rotation [26] , [27] , [28] , [29] , [30] , [31] , [32] , [33] (Fig. 1c ). It can be imagined that (1) if an atom of the stereogenic axis of the diastereomeric intermediates in DyKAT changes from sp 2 to sp 3 under the action of additional reagents, the group on the stereogenic axis may be easier to rotate; (2) if the conversion from sp 2 to sp 3 is reversible, it might be a new model for the interconversion of diastereomeric intermediates in DyKAT. As a result of our continuous interest in tetracoordinate boron chemistry [34] , we envisioned that the reversibility between B( sp 2 ) and B( sp 3 ) [35] , [36] , [37] , [38] , [39] , [40] could support B( sp 3 )-directed DyKAT and fabricate optically pure C-B axially chiral molecules [41] , [42] (Fig. 1d ), which as elusive atropisomers and this type of chiral organoborons are underdeveloped and represent a big hurdle and challenge in boron chemistry as well as in axial chirality compared to their congeners with C-C or C-N axis, owing to the lower rotational barrier which is caused by longer C-B bond [43] , [44] , [45] , [46] , [47] . If successful, this reaction would develop an interesting diastereomeric intermediate equilibrium process that differs from previous chelation-directed DyKAT of racemic heterobiaryls [18] , [19] , [20] , [21] , [22] , [23] , [24] , [25] . Herein, we present a palladium-catalyzed dynamic kinetic asymmetric cross-coupling of racemic, configurationally stable 3-bromo-2,1-azaborines [48] , [49] , [50] , [51] , [52] , [53] with boronic acid derivatives via an equilibrium mode of DyKAT mediated by tetracoordinate boron intermediates. By doing so, the DyKAT strategy could be employed to the assembly of challenging atropisomers with C-B axis or adjacent C-B and C-C diaxes. On the basis of the previous reports of DyKAT [2] , [7] and asymmetric Suzuki−Miyaura coupling reactions [54] , [55] , [56] , [57] , [58] , [59] , [60] , [61] , [62] , [63] , [64] , [65] , [66] , [67] , our proposed catalytic DyKAT version is shown in Fig. 1d . Oxidative addition of racemic 3-bromo-2,1-azaborines to chiral Pd(0) species and subsequent anion exchange afford diastereomeric intermediate I . The fast equilibration of intermediate ( R )-I and ( S )-I could occur through the tetracoordinate boron intermediate II formed by the transfer of the hydroxy group from Pd [68] . Then, the transmetalation between intermediate I and boronic acid derivatives and final reductive elimination generates C-B axial chirality and regenerates the chiral Pd(0) catalysis. It is important that one of the diastereomeric intermediate I ( ( R )-I or ( S )-I ) undergoes the transmetalation step faster than the other, so as to achieve the goal of DyKAT. Although mechanistically appealing, there are several considerable challenges: (1) the sterically hindered environment around B atom may inhibit the formation of tetracoordinate boron intermediates; (2) it is still uncertain whether the tetracoordinate boron intermediate could really reduce the rotation barrier and facilitate rotation of the aryl group on B atom around the C-B stereogenic axis; (3) competitive intramolecular self-coupling side reactions might occur [69] ; (4) the simultaneous diastereoselective and enantioselective synthesis of axially chiral molecules with multiple axes by one-step reactions is still in its infancy [70] , [71] , [72] , [73] , [74] . To validate our hypothesis, we first designed and synthesized racemic 3-bromo-2,1-borazaronaphthalene 1a . Preliminary density functional theory (DFT) calculations were performed to evaluate the feasibilities of the racemization processes of three different species. As depicted in Fig. 2a , substrate 1a with a C–B axis has a rotation barrier of 31.8 kcal/mol to 1a’ since the congested steric environment of the planar geometry in transition states induces large distortions of aromatic rings. Compared with 1a , substrate 1a-C for the traditional asymmetric Suzuki-Miyaura coupling possesses not only a shorter C–C axis but also stronger aromaticity, which renders a much higher rotational barrier of 47.8 kcal/mol to 1a-C’ , making direct dynamic kinetic asymmetric transformation from the substrate (DyKAT) even more unattainable (Fig. 2b ). However, the Lewis acidic boronic complex 1a-Pd , the intermediate after oxidative addition of 1a to Pd followed by ligand exchange, allows the coordination of the hydroxide ligand to form a chiral tetracoordinate boron species. In TS-Pd , the tetracoordinate boron species own elongated C–B axis. The corresponding rotational barrier from 1a-Pd to 1a-Pd’ is significantly reduced to 16.7 kcal/mol (Fig. 2c ), which makes the free rotation of the aryl group around C–B stereogenic axis feasible and fully supports our conjecture. Fig. 2: Preliminary density functional theory (DFT) calculations on the racemization processes and condition optimization. a Activation energy barrier for axial rotation of 3-bromo-2,1-borazaronaphthalene 1a . b Activation energy barrier for axial rotation of 3-bromo-naphthalene 1a-C . c Activation energy barrier for axial rotation of 3-Pd-2,1-borazaronaphthalene via a TS featuring tetracoordinate boron geometry, TS-Pd . d Condition optimization for palladium-catalyzed dynamic kinetic asymmetric cross-coupling. Full size image Encouraged by the results from theoretical calculations, we then investigated this envisioned dynamic kinetic cross-coupling using racemic 3-bromo-2,1-borazaronaphthalene 1a and trifluoroborate 2a as model substrates (Fig. 2d ). Delightfully, this reaction with Pd 2 (dba) 3 as catalyst, the P-chiral monophosphorus ligand L1 as ligand and Cs 2 CO 3 as base in toluene/H 2 O furnished the desired C-B axially chiral product ( R )-3a in 81% NMR yield with 25% enantioselectivity excess (ee) at 40 °C (Fig. 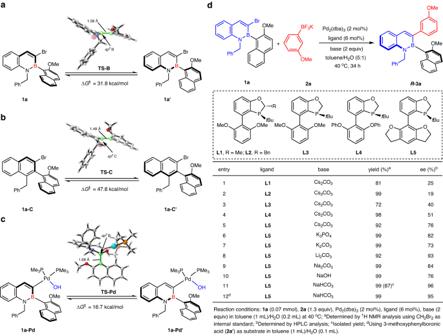Fig. 2: Preliminary density functional theory (DFT) calculations on the racemization processes and condition optimization. aActivation energy barrier for axial rotation of 3-bromo-2,1-borazaronaphthalene1a.bActivation energy barrier for axial rotation of 3-bromo-naphthalene1a-C.cActivation energy barrier for axial rotation of 3-Pd-2,1-borazaronaphthalene via a TS featuring tetracoordinate boron geometry,TS-Pd.dCondition optimization for palladium-catalyzed dynamic kinetic asymmetric cross-coupling. 2d , entry 1). This result proved the feasibility of our hypothesis and encouraged us to further evaluate other ligands. The P-chiral monophosphorus ligands with small steric hindrance led to higher ee values (Fig. 2d , entries 1–3). The substituents on the aryl units of the ligands have an effect on this reaction (Fig. 2d , entries 4-5), and a better result (Fig. 2d , entry 5, 92% yield and 76% ee) was obtained when ligand L5 with tetrahydrobenzofuran group was used. Subsequently, we investigated the effect of bases and found that these bases all promoted this reaction well, but the enantioselectivities of this reaction were sensitive to bases (Fig. 2d , entries 6–10). In general, weak bases were more favorable for enantioselectivities than strong bases. Overall, the optimized reaction conditions for this DyKAT are shown below: 1a (1 equiv), 2a (1.3 equiv), Pd 2 (dba) 3 (2 mol%), L5 (6 mol%), NaHCO 3 (2 equiv) in toluene/H 2 O at 40 °C for 34 h (Fig. 2d , entry 11). In addition, the same yield and enantioselectivity were obtained by reducing the proportion of water when 3-methoxyphenylboronic acid ( 2a’ ) was used as the substrate (Fig. 2d , entry 12). To better understand the racemization process of the DyKAT, the following experiments were performed. As illustrated in Fig. 3a , the profile of the ee values or yields of the recovered 1a and the product 3a versus time indicated that two enantiomers of 1a were consumed together and one of the enantiomers was decreased more rapidly, suggesting a kinetic resolution (KR) process. In addition, the reactions of enantioenriched 1a (37% ee) with two ligands with different configurations were carried out, and the profile of the ee values of the recovered 1a versus time was shown in Fig. 3b . The results also supported a KR process. Finally, no obvious racemization of enantioenriched 3-bromo-2,1-azaborine 1a under standard conditions without aryl trifluoroborates, excluding a dynamic kinetic resolution (DKR) pathway. To demonstrate that the process is indeed a DyKAT, DFT calculations were performed to probe the mechanism of the racemization process. After oxidative addition and anion ligand exchange, benefiting from the boron Lewis acidity, IM0 first underwent an intramolecular hydroxide migration to form a tetracoordinate boron species IM1 via TS1 . The C-B bond in IM1 is free to rotate with a small barrier of 5.2 kcal/mol. The analysis of the geometry of TS2 indicates that owing to the formation of tetracoordinate structure, the naphthalene moiety undergoing rotation is placed on the axial position to avoid repulsions with the benzylic group sprouted on the equatorial position. Meanwhile, the C–B bond is elongated by ~0.1 Å, which also provides more space to relax the strain in TS2 . Interestingly, IM2 is more stable than its diastereomer IM1 due to the formation of an intramolecular hydrogen bond. The overall energy barrier for the racemization process is 13.8 kcal/mol, endorsing our strategy that the rotation around C–B axis could be realized even with very bulky ligands. Fig. 3: Mechanistic studies. a Yields and ee values of product 3a (recovered 1a ) at different reaction times. b Ee values of recovered 1a at different reaction times by using ligands L5 and (-)-L5 . c Racemization experiment under standard conditions without aryl trifluoroborates. d Free energy profile calculated for the racemization process with L5 as ligand. Full size image Applying the optimized reaction conditions to a range of substrates demonstrates the generality of this DyKAT (Fig. 4 ). This approach was compatible with aryl trifluoroborate bearing electron-rich groups, including alkoxy ( 3a, 3b , and 3e – 3j ), methylthio ( 3c ), and N , N -diphenyl ( 3d ), delivering the corresponding C-B axially chiral products in high yields with good to excellent enantioselectivities (80–96% ee). The absolute configuration of ( R a )-3a was determined by X-ray crystallographic analysis (CCDC 2245394, the CIF file is provided in Supplementary Data 1 ). Aryl trifluoroborate with an electron-withdrawing group was tolerated well under the standard conditions ( 3k , 70% yield and 93% ee). The tetrastyryl group could also be introduced into the desired product 3l by this method, which provides the possibility for a chiral AIE molecule. Polycyclic aryl trifluoroborates ( 3m and 3n ) and unsubstituted phenyl trifluoroborate ( 3q ) were successfully coupled with excellent enantioselectivities to desired products. Moreover, aryl trifluoroborates bearing heteroaromatic components, including carbazoles ( 3o and 3p ), furan ( 3r ), thiophene ( 3s ), and benzothiophene ( 3t ), could be smoothly converted into the target products with good to excellent enantioselectivities (82–96% ee). Alkenyl trifluoroborates underwent this reaction well, and the better enantioselectivities of 1-substituted alkenyl trifluoroborates ( 3v and 3w ) than ( E )-styryl trifluoroborate ( 3u ) may be due to steric hindrance. Fig. 4: Substrate scope for trifluoroborates. Reaction conditions: 1 (0.1 mmol), 2 (0.13 mmol), Pd 2 (dba) 3 (2 mol%), L5 (6 mol%), NaHCO 3 (2 equiv) in toluene (1.5 mL)/H 2 O (0.3 mL) at 40 °C; isolated yields are provided. Full size image Next, a wide range of racemic 3-bromo-2,1-borazaronaphthalenes could all undergo this DyKAT to render the corresponding enantiomerically enriched C-B axially chiral molecules (Fig. 5a ). Methoxy ( 3x ), methyl ( 3 y and 3ah ), and fluoro ( 3z )-substituted racemic 3-bromo-2,1-borazaronaphthalenes could successfully deliver the desired products in excellent efficiency (77–98% yields and 96–98% ee). 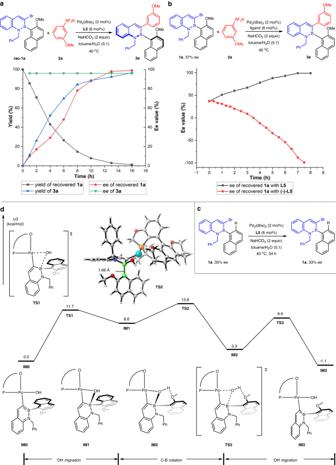Fig. 3: Mechanistic studies. aYields and ee values of product3a(recovered1a) at different reaction times.bEe values of recovered1aat different reaction times by using ligandsL5and(-)-L5.cRacemization experiment under standard conditions without aryl trifluoroborates.dFree energy profile calculated for the racemization process withL5as ligand. Notably, BN-phenanthrene ( 3aa ) was a viable framework for this transformation, providing the corresponding product with excellent enantioselectivity. Moreover, substituents on the N atom of the 2,1-borazaronaphthalene including benzyls ( 3ab - 3ad ), n -butyl ( 3ae ), and thiophen-2-ylmethyl ( 3af ) were readily tolerated well. Despite lower yield, the transformation also tolerated bulky (isopropyl) moiety on the N atom of the 2,1-borazaronaphthalene with excellent enantioselectivity ( 3ag , 33% yield and 97% ee). Low enantioselectivities were obtained when the OMe group was changed to the OEt ( 3ai ) or SEt ( 3aj ) groups with larger steric hindrance. Fig. 5: Substrate scope for racemic 3-bromo-2,1-borazaronaphthalenes and diaxially chiral compounds. a Scope for racemic 3-bromo-2,1-borazaronaphthalenes. Reaction conditions: 1 (0.1 mmol), 2a (0.13 mmol), Pd 2 (dba) 3 (2 mol%), L5 (6 mol%), NaHCO 3 (2 equiv) in toluene (1.5 mL)/H 2 O (0.3 mL) at 40 °C; isolated yields are provided. b Scope of adjacent C-B and C-C diaxially chiral compounds. Reaction conditions: 1 (0.1 mmol), 2-methoxy-1-naphthyl)boronic acid (1.3–4.0 equiv), Pd 2 (dba) 3 (2 mol%), L5 (6 mol%), Li 2 CO 3 (2.0–4.0 equiv) in toluene (1.5 mL)/H 2 O (0.15 mL) at 40 °C; isolated yields are provided. Full size image In view of the successful application of the DyKAT strategy to prepare the C-B axially chiral compounds, we turned our attention to the synthesis of atropisomers with C-B adjacent diaxes of C-B and C-C bonds (Fig. 5b ). (2-Methoxy-1-naphthyl)boronic acid was tested in the reaction, and to our delight, the desired axially chiral products 3ak - 3an were obtained with excellent diastereoselectivities and enantioselectivities (>20:1 dr, 95–97% ee). The absolute configuration of 3ak was determined by ECD and two-dimensional NMR experiments (for details, see Supplementary Figs. 1 – 4 and 6 – 10 ) [75] , [76] , [77] . This transformation is also applicable to the synthesis of C-B axially chiral compounds bearing complex fragments derived from natural products or therapeutic agents, whose high functional-group compatibility is fully linchpinned. Aryl trifluoroborates derived from clofibrate ( 4a ), estrone ( 4b ), and tyrosine ( 4c ) were transformed into the corresponding C-B axially chiral compounds with ease (Fig. 6a ). In addition, C-B axially chiral compounds could be further modified. Firstly, demethylation of product 3 m could generate a C-B axially chiral molecule 5 with free naphthol, which has the potential for further transformations (Fig. 6b ). Meanwhile, product 3 u could be converted to isopropyl-substituted C-B axially chiral molecule 6 via hydrogenation, and could also react with indole under acid catalysis to afford compound 7 with high retention of the enantiopurity (Fig. 6c ). Fig. 6: Functionalization of complex molecules and synthetic transformations. a Functionalization of complex molecules. b Demethylation of 3m . c Palladium-catalyzed hydrogenation of 3u and Brønsted acid-catalyzed alkylation of indole with 3u as alkylation reagent. Boc = t -butoxycarbonyl. Full size image In conclusion, we developed a palladium-catalyzed DyKAT process of racemic, configurationally stable 3-bromo-2,1-azaborines for the construction of C-B axial chirality. The experiments and calculations demonstrated that the reaction is a DyKAT process and that the reversible tetracoordinate boron intermediate is the key to its success. This chemistry offers practical access to chiral organoborons bearing C-B axis or adjacent C-B and C-C diaxes in generally high yields with excellent diastereoselevtivities and enantioselctivities. General procedure for the synthesis of atropisomers with a single C-B stereogenic axis In air, a 25 mL Schlenk tube was charged with 1 (0.1 mmol, 1 equiv), 2 (0.13 mmol, 1.3 equiv), Pd 2 (dba) 3 (2 mol%), L5 (6 mol%), and NaHCO 3 (0.2 mmol, 2.0 equiv). The tube was evacuated and filled with argon for three cycles. Then, 1.5 mL of toluene and 0.3 ml of water was added under argon. The reaction was allowed to stir at 40 °C for 34 h. Upon completion, a proper amount of silica gel was added to the reaction mixture. After the removal of the solvent, the crude reaction mixture was purified on silica gel (petroleum ether and ethyl acetate) to afford the desired products. 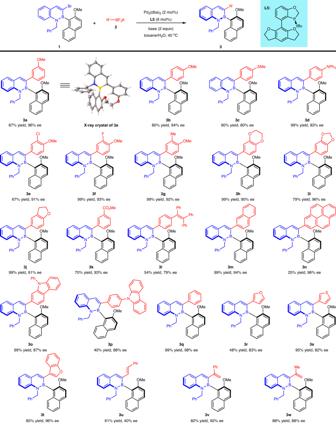Fig. 4: Substrate scope for trifluoroborates. Reaction conditions:1(0.1 mmol),2(0.13 mmol), Pd2(dba)3(2 mol%),L5(6 mol%), NaHCO3(2 equiv) in toluene (1.5 mL)/H2O (0.3 mL) at 40 °C; isolated yields are provided. General procedure for the synthesis of atropisomers with adjacent diaxes of C-B bond and C-C bond In air, a 25 mL Schlenk tube was charged with 1 (0.1 mmol, 1 equiv), 2-methoxy-1-naphthyl)boronic acid (1.3–4.0 equiv), Pd 2 (dba) 3 (2 mol%), L5 (6 mol%), and Li 2 CO 3 (2.0–4.0 equiv). The tube was evacuated and filled with argon for three cycles. 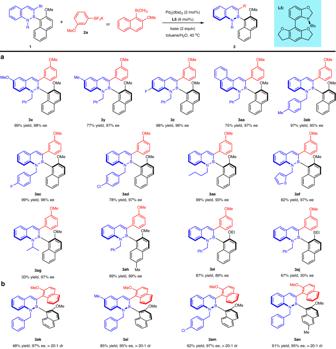Fig. 5: Substrate scope for racemic 3-bromo-2,1-borazaronaphthalenes and diaxially chiral compounds. aScope for racemic 3-bromo-2,1-borazaronaphthalenes. Reaction conditions:1(0.1 mmol),2a(0.13 mmol), Pd2(dba)3(2 mol%),L5(6 mol%), NaHCO3(2 equiv) in toluene (1.5 mL)/H2O (0.3 mL) at 40 °C; isolated yields are provided.bScope of adjacent C-B and C-C diaxially chiral compounds. Reaction conditions:1(0.1 mmol), 2-methoxy-1-naphthyl)boronic acid (1.3–4.0 equiv), Pd2(dba)3(2 mol%),L5(6 mol%), Li2CO3(2.0–4.0 equiv) in toluene (1.5 mL)/H2O (0.15 mL) at 40 °C; isolated yields are provided. 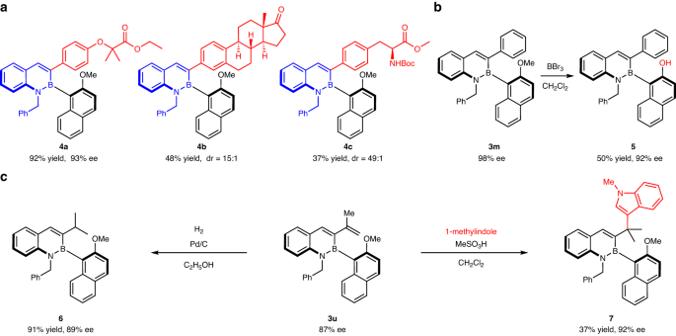Fig. 6: Functionalization of complex molecules and synthetic transformations. aFunctionalization of complex molecules.bDemethylation of3m.cPalladium-catalyzed hydrogenation of3uand Brønsted acid-catalyzed alkylation of indole with3uas alkylation reagent. Boc =t-butoxycarbonyl. Then, 1.5 mL of toluene and 0.15 ml of water was added under argon. The reaction was allowed to stir at 40 °C for 46–76 h. Upon completion, a proper amount of silica gel was added to the reaction mixture. After the removal of the solvent, the crude reaction mixture was purified on silica gel (petroleum ether and ethyl acetate) to afford the desired products.